Enantioselective synthesis of a chiral nitrogen-doped buckybowl Bowl-shaped aromatic compounds, namely buckybowls constitute a family of curved polycyclic aromatic carbons along with fullerenes and carbon nanotubes. Doping of heteroatoms to the carbon frameworks of such aromatic compounds drastically modulates their physical and chemical properties. In contrast to nitrogen-doped azafullerenes or carbon nanotubes, synthesis of azabuckybowls, nitrogen-doped buckybowls, remains an unsolved challenging task. Here we report the first enantioselective synthesis of a chiral azabuckybowl, triazasumanene. X-ray crystallographic analysis confirmed that the doping of nitrogen induces a more curved and deeper bowl structure than in all-carbon buckybowls. As a result of the deeper bowl structure, the activation energy for the bowl inversion (thermal flipping of the bowl structure) reaches an extraordinarily high value (42.2 kcal per mol). As the bowl inversion corresponds to the racemization process for chiral buckybowls, this high bowl inversion energy leads to very stable chirality of triazasumanene. Polycyclic aromatic carbons with curved π -conjugated structures, such as fullerenes and carbon nanotubes (CNTs), exhibit fascinating physicochemical properties especially in material science [1] , [2] , [3] . Chemical doping of heteroatoms to the lattice of the carbon frameworks is an effective strategy to modulate their intrinsic physical and chemical properties [4] , [5] . In particular, among the potential dopants, nitrogen is considered to be one of the more fascinating elements for chemical doping. Aza[60]fullerene C 59 N and its dimer are the most studied heterofullerenes [6] . Nitrogen-containing CNTs and graphene exhibit fascinating and unique properties [7] , [8] , [9] . Buckybowls, bowl-shaped aromatic hydrocarbons, are known as fullerene fragments or the cap structures of CNTs, which constitute a family of curved aromatic compounds with fullerenes and CNTs. Buckybowls have attracted much attention not only as model compounds for fullerenes, but also for their own chemical and physical properties [10] , [11] , [12] , [13] . In contrast to nitrogen-doped fullerenes and CNTs, nitrogen-doped buckybowls, azabuckybowls, still remain unknown except for some theoretical studies [14] , [15] . Doping of nitrogen to the aromatic skeleton is expected to modulate the curvature, bowl inversion barrier, and physicochemical properties. Heterobuckybowls doped by larger heteroatoms other than carbon such as S, Si and Sn exhibited less curvature, resulting in shallower bowls or planar structures [16] , [17] , [18] . In contrast, azabuckybowls doped by nitrogen atoms, which are smaller than carbon atoms, are predicted by calculations to exhibit more curvature with deeper bowl depth than all-carbon bowls [14] . Synthesis of such a highly strained bowl structure has been a challenging task for a long time [19] . Buckybowls are expected to be potential precursors for fullerenoids or CNTs by elongation of the aromatic frameworks [20] , [21] . Therefore, organic synthesis of azabuckybowls to control the position of nitrogen atoms and their chirality is considered to be important not only for their own properties but also for the development of related curved aromatic compounds. Triazasumanene is a C 3 -symmetric azabuckybowl, where three nitrogen atoms are doped in sumanene [22] ( Fig. 1a ). Triazasumanenes possess 'bowl chirality' [23] , [24] , [25] ( Fig. 1b ), which derives from their three-dimensional geometry (for the nomenclature of chiral buckybowls, see Supplementary Methods ). In this study, we develop an enantioselective synthesis of triazasumanene (R=SMe) 1 by controlling the bowl chirality. Our synthetic strategy involves construction of the three-dimensional bowl framework using tetrahedral sp 3 carbons, leading to the required π -conjugated structure by oxidative aromatization; and transmission of sp 3 stereogenic centres to bowl chirality. Mild-reaction conditions in the solution-phase enable the control of the high reactivity derived from nitrogen atoms as well as the transmission of chirality. By this strategy, we achieved the first enantioselective synthesis of a nitrogen-doped azabuckybowl, triazasumanene [26] . 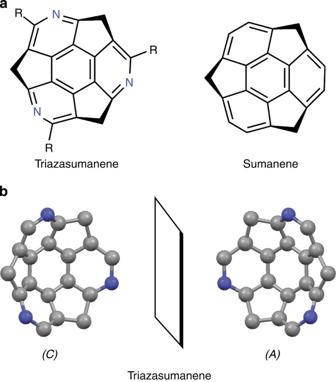Figure 1: Structures of sumanene and triazasumanenes. (a) Triazasumanene and sumanene. (b) Enantiomers of triazasumanene. For the nomenclature of chiral buckybowls, seeSupplementary Methods. Figure 1: Structures of sumanene and triazasumanenes. ( a ) Triazasumanene and sumanene. ( b ) Enantiomers of triazasumanene. For the nomenclature of chiral buckybowls, see Supplementary Methods . Full size image Synthesis of triazasumanenes The synthesis is shown in Fig. 2 . Enantiopure (1 S , 4 R )- 2 was converted to syn - 3 exclusively under Pd-catalysed cyclotrimerization conditions [27] . Compound 3 was hydrolysed, followed by condensation, to afford the non-conjugated bowl-shaped lactam 4 . Many attempts to transform 4 directly to aromatic bowl-shaped triazasumanene were unsuccessful. Thus, it was converted to thioimidate 5 by a microwave-assisted thiation reaction utilizing Lawesson's reagent, deprotection of PMB, and treatment with MeI. Dehydrogenation of thioimidate 5 was successfully achieved by combination of Ph 3 CBF 4 as an oxidant and a sterically hindered non-nucleophilic base DTBMP as an acid scavenger [28] to afford ( C )-(−)- 1 in 73% yield after optimization ( Supplementary Tables S1 and S2 ). The opposite enantiomer ( A )-(+)- 1 was similarly prepared from (1 R , 4 S )- 2 . Unfortunately, a single crystal of 1 for the X-ray crystallographic analysis was not obtained to confirm the structure. However, 1 was oxidized by m -CPBA to afford sulfone 6 , which gave single crystals suitable for X-ray crystallographic analysis. 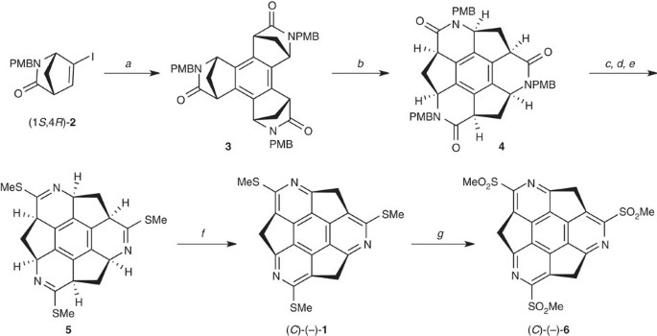Figure 2: Enantioselective synthesis of triazasumanenes 1 and 6. Conditions:a. Pd(OAc)2, PPh3, Bu4NOAc, Na2CO3, molecular sieves 4 Å, 1,4-dioxane, 100 °C, 2 h, 57%;b. (i) 12 M HCl, AcOH, 60 °C, 3 h; (ii) C6F5OP(=O)Ph2,N,N-diisopropylethylamine, DMF, 0 to 60 °C, 59% (two steps);c. Lawesson's reagent, 1,2-dichloroethane, microwave, 160 °C, 40 min, 92%;d. Trifluoroacetic acid, microwave, 100 °C, 2 h, 88%;e. MeI, K2CO3, DMF, 30 °C, 3 h, 79%;f. Ph3CBF4, DTBMP, CH2Cl2, 25 °C, 8 h, 73%;g.m-CPBA, CH2Cl2, 0 °C then 15 °C 2 h, 90%. PMB,p-MeOC6H4CH2; DMF,N,N-dimethylformamide; DTBMP, 2,6-di-tert-butyl-4-methyl- pyridine; Lawesson's reagent, 2,4-bis(4-methoxyphenyl)-1,3,2,4-dithiadiphosphetane-2,4-disulfide;m-CPBA, 3-chloroperoxybenzoic acid. Figure 2: Enantioselective synthesis of triazasumanenes 1 and 6. Conditions: a . Pd(OAc) 2 , PPh 3 , Bu 4 NOAc, Na 2 CO 3 , molecular sieves 4 Å, 1,4-dioxane, 100 °C, 2 h, 57%; b . (i) 12 M HCl, AcOH, 60 °C, 3 h; (ii) C 6 F 5 OP(=O)Ph 2 , N , N -diisopropylethylamine, DMF, 0 to 60 °C, 59% (two steps); c . Lawesson's reagent, 1,2-dichloroethane, microwave, 160 °C, 40 min, 92%; d . Trifluoroacetic acid, microwave, 100 °C, 2 h, 88%; e . MeI, K 2 CO 3 , DMF, 30 °C, 3 h, 79%; f . Ph 3 CBF 4 , DTBMP, CH 2 Cl 2 , 25 °C, 8 h, 73%; g . m- CPBA, CH 2 Cl 2 , 0 °C then 15 °C 2 h, 90%. PMB, p -MeOC 6 H 4 CH 2 ; DMF, N , N -dimethylformamide; DTBMP, 2,6-di- tert -butyl-4-methyl- pyridine; Lawesson's reagent, 2,4-bis(4-methoxyphenyl)-1,3,2,4-dithiadiphosphetane-2,4-disulfide; m -CPBA, 3-chloroperoxybenzoic acid. Full size image X-ray crystallography The nitrogen-doped aromatic bowl structure was confirmed by the X-ray crystallographic analysis of ( C )-(−)- 6 ( Supplementary Data 1 ). The packing structure and ORTEP drawings of a single molecule of ( C )-(−)- 6 are illustrated ( Fig. 3a–d ; Supplementary Figs S1 and S2 ). The packing structure adopts a quasi convex–convex and concave–concave stacking model. While the pyridine rings are stacked at the convex–convex faces with an centroid-to-centroid distance of 3.88 Å ( Fig. 3a , red dashed line), the interaction of the oxygen atom of the sulfonyl groups and the central benzene rings are observed at both concave and convex faces of the central benzene rings with 2.78–3.59 Å distances ( Fig. 3a , blue dashed lines). The bowl depth is measured as 1.30 Å based on the rim nitrogen atoms ( Fig. 3d ), which is deeper than that of sumanene (1.11 Å) [29] ( Supplementary Fig. S2 ). Haddon's π -orbital axis vector (POAV) analysis [30] ( Fig. 3e ) reveals that the six hub carbons are pyramidalized to an extent of 10.0° for C1 and 10.7° for C2 ( Fig. 3e ), both of which are bigger than sumanene (9.0°) [29] , and the latter is comparable to that of hemifullerene C 30 H 12 (10.8°) [31] . 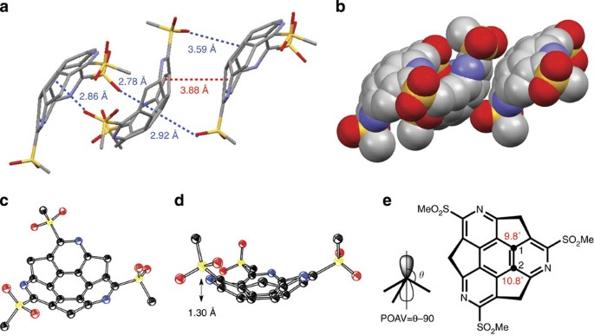Figure 3: X-ray crystallographic analysis of compound (C)-(−)-6. All hydrogen atoms were omitted for clarity. (a) Packing model of (C)-6(blue lines: distance between oxygen atoms of sulfonyl groups and centroid of central benzene rings; red lines, centroid-to-centroid distance between two pyridine rings). (b) Spacefilling drawings of packing of (C)-6. (c) ORTEP drawings of (C)-6: top view (with thermal ellipsoids set at 50% probability). (d) Side view with bowl depth. (e) Haddon'sπ-orbital axis vector (POAV angle)30and POAV angles of (C)-6. Figure 3: X-ray crystallographic analysis of compound ( C )-(−)-6. All hydrogen atoms were omitted for clarity. ( a ) Packing model of ( C )- 6 (blue lines: distance between oxygen atoms of sulfonyl groups and centroid of central benzene rings; red lines, centroid-to-centroid distance between two pyridine rings). ( b ) Spacefilling drawings of packing of ( C )- 6 . ( c ) ORTEP drawings of ( C )- 6 : top view (with thermal ellipsoids set at 50% probability). ( d ) Side view with bowl depth. ( e ) Haddon's π -orbital axis vector (POAV angle) [30] and POAV angles of ( C )- 6 . Full size image Bowl inversion and chirality One interesting property of buckybowls is their dynamic bowl inversion [32] , which is the thermal flipping of the bowl structure through a flat transition structure ( Fig. 4a ). For example, a C 5 -symmetric buckybowl, corannulene (C 20 H 10 ), has a bowl inversion energy of ΔG ‡ =11.5 kcal per mol and exhibits rapid bowl inversion at room temperature (>20,000 times per second) [33] , whereas the bowl inversion energy of sumanene is ΔG ‡ =20.3 kcal per mol and the inversion is much slower (one time per 143 s) [34] . For a chiral buckybowl possessing bowl chirality, the bowl inversion corresponds to the racemization process ( Fig. 4a ). We have previously reported the first enantioselective synthesis of a chiral buckybowl, trimethylsumanene [23] . However, it undergoes quick racemization at 20 °C ( t 1/2 =23 min) because of the relatively low bowl inversion energy (ΔG ‡ =21.6 kcal per mol). In contrast, triazasumanenes were expected to possess higher bowl inversion energies because of the deeper bowl structure, as a result of the doping effect of the nitrogen atoms. The bowl inversion energy of 1 was estimated by density functional theory calculations (B3LYP/6-311+G(d,p)) to be ΔE=39.9 kcal per mol ( Supplementary Figs S3 and S4 ; Supplementary Tables S3 and S4 ), which corresponds to 1.1 billion years for a half-lifetime at 20 °C, whereas the calculated values for sumanene and trimethylsumanene are ΔE=18.3 kcal per mole and 19.2 kcal per mole, respectively [25] . Indeed, enantiomeric excesses (ee) of both enantiomers of enantioselectively prepared 1 were determined to be >99% by chiral high-performance liquid chromatography (HPLC) analysis at room temperature. The circular dichroism (CD) spectra of 1 ( Fig. 4b ) and 6 ( Supplementary Fig. S5 ) were recorded at room temperature and no decay was observed after 1 week. These results strongly indicate that compound 1 and 6 should have much higher bowl inversion energy and it should not racemize at room temperature. According to the calculated value, we tried to observe the racemization of 1 at high temperature and determine the bowl inversion/racemization energy experimentally ( Fig. 4c,d ). Thus, a solution of enantiopure ( C )-(−)- 1 in anhydrous tetralin was heated at 488 K under inert atmosphere and the sample was analysed by chiral HPLC. After 12–84 h, the gradual formation of the other enantiomer was observed without decomposition ( Fig. 4c ). From the racemization experiment, the rate constant and bowl inversion/racemization energy (ΔG ‡ ) of 1 were determined to be 1.24×10 −6 s −1 (488 K) and 42.2 kcal per mole according to the Eyring equation ( Fig. 4d ), respectively, which corresponds to 54 billion years for the half-lifetime at 20 °C. Thus, the extraordinarily high bowl inversion energy and the stable bowl chirality were experimentally proven as well. The stable bowl chirality of triazasumanene is distinct in contrast to the quick racemization of chiral sumanene derivatives with all-carbon frameworks. 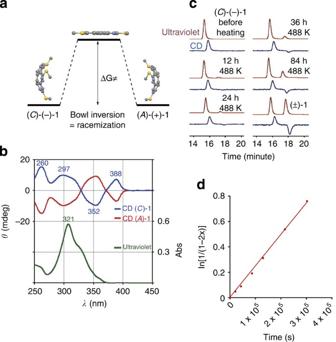Figure 4: Chirality and bowl inversion energy. (a) Representation of bowl inversion of compound1. For chiral compounds, this inversion process corresponds to racemization. The inversion energy ΔG≠can be determined by kinetic measurement of the rate constant of the racemic process through the Eyring equation. (b) CD and ultraviolet/visible spectra of compound1in CH2Cl2solution (1.2×10−5M). Blue line and red line are CD spectra of (C)-(−)-1and (A)-(+)-1, respectively. Green line is ultraviolet/visible spectrum. (c) Chiral HPLC traces of the racemization process of compound (C)-(−)-1(racemization was carried out at 488 K for the time indicated on the charts (before heating, enantiopure (C)-(−)-1, >99% ee; 12 h; 24 h; 36 h; 84 h); HPLC analysis was performed at 263 K on a Daicel Chiralpak IA column); racemic sample was obtained by mixture (C)-(−)-1and (A)-(+)-1in 1:1 ratio. (d) Plot of ln[1/(1−2x)] versus t (s), x is the concentration of newly generated (A)-(+)-1at time t. A linear curve fitting equation: y=2.48×10−6x,R2=0.998. Rate constantk=1.24×10−6s−1. Figure 4: Chirality and bowl inversion energy. ( a ) Representation of bowl inversion of compound 1 . For chiral compounds, this inversion process corresponds to racemization. The inversion energy ΔG ≠ can be determined by kinetic measurement of the rate constant of the racemic process through the Eyring equation. ( b ) CD and ultraviolet/visible spectra of compound 1 in CH 2 Cl 2 solution (1.2×10 −5 M). Blue line and red line are CD spectra of ( C )-(−)- 1 and ( A )-(+)- 1 , respectively. Green line is ultraviolet/visible spectrum. ( c ) Chiral HPLC traces of the racemization process of compound ( C )-(−)- 1 (racemization was carried out at 488 K for the time indicated on the charts (before heating, enantiopure ( C )-(−)- 1 , >99% ee; 12 h; 24 h; 36 h; 84 h); HPLC analysis was performed at 263 K on a Daicel Chiralpak IA column); racemic sample was obtained by mixture ( C )-(−)- 1 and ( A )-(+)- 1 in 1:1 ratio. ( d ) Plot of ln[1/(1−2x)] versus t (s), x is the concentration of newly generated ( A )-(+)- 1 at time t. A linear curve fitting equation: y=2.48×10 −6 x, R 2 =0.998. Rate constant k= 1.24×10 −6 s −1 . Full size image The first nitrogen-doped chiral buckybowls 1 and 6 were enantioselectively synthesized. The X-ray crystallographic analysis of compound 6 confirmed that the doping of nitrogen leads to a more curved and deeper bowl, which is extraordinary for a buckybowl of such a small size. As a result of the deeper bowl structure, the activation energy for the bowl inversion reaches an extraordinarily high value (42.2 kcal per mole). As the bowl inversion corresponds to the racemization process for chiral buckybowls, this high bowl inversion energy leads to the very stable chirality. Our study demonstrates that the doping of nitrogen atoms to buckybowls drastically change the structural and physicochemical properties of buckybowls. As buckybowls constitute a class of curved aromatic compounds of growing interest as materials, for their structural variability and synthetic availability, we envisage that rational incorporation of nitrogen and other heteroatoms into the aromatic framework of buckybowls will be a general and effective strategy to modulate their physicochemical and electronic properties. Materials and characterization Microwave reactions were carried out on a Biotage Initiator microwave reactor in sealed microwave process vials. Melting points were determined on an automated melting point system and were uncorrected. 1 H and 13 C NMR spectra were recorded on a JEOL JNM-LA400 spectrometer at 400 and 100 MHz, respectively. High resolution mass spectra (HRMS) were measured using electron impact mode (EI) methods. Chiral HPLC analysis was performed using Ultraviolet/visible and CD detectors. CD spectra were recorded on JASCO J-720WI spectropolarimeter. Ultraviolet spectra were measured on a JASCO V-670 spectrometer. Infrared spectra (IR) were recorded on a JASCO FT/IR 4100 spectrometer. Silica gel chromatography was performed on neutral silica gel using a preparative medium pressure liquid chromatography system. For thin-layer chromatography (TLC) analysis throughout this work, Merck pre-coated TLC plates (silica gel 60 F254 0.25 mm) were used. For preparative thin-layer chromatography, Merck pre-coated PLC plates (silica gel 60 F254, 0.5 mm) were used. Air- and/or moisture-sensitive reactions were carried out under argon atmosphere with anhydrous solvents. Anhydrous solvents were used as received. Other reagents were used as received without further purification. Both enantiomers of compound 2 and compound 3 were prepared according to our reported method [27] . Preparation and characterization of compound 5 from compound 3 are included in Supplementary Methods and Supplementary Figs S6–S9 . Synthesis of compounds ( C )-9,14,19-tris(methylthio)-8,13,18-triazasumanene 1 . To a solution of compound 5 (41 mg, 0.10 mmol) and DTBMP (164 mg, 0.80 mmol) in anhydrous CH 2 Cl 2 (30 ml) was added Ph 3 CBF 4 (200 mg, 0.60 mmol) under Ar atmosphere. The mixture was stirred at 25 °C for 8 h, during which the colour changed from yellow to dark red. The completion of reaction was determined by 1 H NMR analysis as follows: 0.5 ml of the mixture was taken out, quenched with aqueous NaHCO 3 , extracted, dried over Na 2 SO 4 , evaporated, and dissolved in CDCl 3 for 1 H NMR analysis. When most of starting material 5 (>95%) was consumed, aqueous NaHCO 3 solution was added to the reaction mixture. The mixture was stirred for 10 minutes. The organic layer was separated and the aqueous layer was extracted with CH 2 Cl 2 (2×15 ml). The combined organic layer was washed with aqueous NaHCO 3 solution and brine successively. The organic layer was dried over Na 2 SO 4 , filtered, and evaporated to give a yellow solid. The crude product was purified by silica gel column chromatography (5% EtOAc/CH 2 Cl 2 ) to afford compound 1 as a white solid, which contained about <5% starting material 5 . As starting material 5 and product 1 show the same R f value by using of EtOAc/CH 2 Cl 2 as eluting solvent, trace amount of starting material can be removed by silica gel chromatography using 5% EtOAc/toluene as eluent or simply washing with EtOAc. Pure triazasumanene 1 was obtained as a white solid (29.6 mg, 73%). [ α ] 21 D : −291.3 ( c =0.25, CHCl 3 ); mp: >280 °C (decomp. ); IR (KBr): ν 2,935, 2,839, 1,724, 1,617, 1,533, 1,405, 1,310, 1,134, 995, 789 cm −1 ; 1 H NMR (400 MHz, CDCl 3 ): δ 4.63 (d, J =19.2 Hz, 3H), 3.08 (d, J =19.2 Hz, 3H), 2.51 (s, 9H); 13 C NMR (100 MHz, CDCl 3 ): δ 175.8, 160.2, 157.5, 139.2, 136.2, 43.4, 13.6 ( Supplementary Fig. S10); HRMS (EI) m/z Calcd for C 21 H 15 N 3 S 3 (M + ): 405.0428; Found: 405.0430. ( C )-9,14,19-tris(methylsulfonyl)-8,13,18-triazasumanene 6 . To a solution of compound 1 (8 mg, 0.02 mmol) in CH 2 Cl 2 (8 ml) cooled to 0 °C was added a solution of m -CPBA (49 mg, 0.20 mmol) in CH 2 Cl 2 (3 ml) in three separated portions at every 1 h. After the addition, the mixture was warmed up to 15 °C for 2 h and TLC showed the consumption of starting material. The reaction was quenched by addition of Me 2 S (20 μl). After stirring for 10 min, to the mixture was added saturated aqueous NaHCO 3 solution and the aqueous solution was extracted with CH 2 Cl 2 (3×10 ml). The combined organic layer was washed with aqueous NaHCO 3 solution and brine, dried over Na 2 SO 4 , and filtered. Evaporation of solvent afforded a white solid quantitatively and 1 H NMR showed that the compound was pure enough (>96% purity). The product was further purified by preparative thin-layer chromatography (MeOH/CH 2 Cl 2 =1/12) to afford pure compound 6 (8.9 mg, 90%). [ α ] 21 D : −543.9 ( c =0.25, CH 2 Cl 2 ); mp: >280 °C (decomp. ); IR (KBr): ν 2,926, 1,632, 1,397, 1,306, 1,143, 957, 756 cm −1 ; 1 H NMR (400 MHz, CD 2 Cl 2 ): δ 5.20 (d, J =19.8 Hz, 3H), 4.05 (d, J =19.8 Hz, 3H), 3.18 (s, 9H); 13 C NMR (100 MHz, CD 2 Cl 2 ): δ 176.4, 161.1, 154.7, 147.9, 142.2, 45.2, 40.9 ( Supplementary Fig. S11 ); HRMS (EI) m/z calcd for C 21 H 15 N 3 O 6 S 3 (M + ): 501.0123; found 501.0116. X-ray crystallography Single crystals were obtained as bright colourless plates (0.5 mm×0.1 mm×0.05 mm) by diffusion of MeOH (1 ml) into a solution of compound ( C )-(−)- 6 (3 mg) in CH 2 Cl 2 (2 ml) at room temperature. Single- crystal X-ray diffraction was performed on a Rigaku Mercury CCD (Mo- Kα , ( λ =0.71073 Å) at 153 K. Data were collected and processed by using Crystal Clear software (Rigaku). The crystallographic details are given in a CIF file ( Supplementary Data 1 ). The crystallographic data of ( C )-(−)- 6 can be obtained free of charge from Cambridge Crystallographic Data Center (CCDC-864009). Crystal data for ( C )-(−)- 6 : monoclinic, space group P21, a =11.295(12), b =14.798 (15), c =12.421 (14) Å, α =90.00, β =101.882(14), γ =90.00°, V =2032(4) Å 3 , Z =4; R 1 =0.0724; wR 2 =0.1091, Flack parameter=0.05(8). Bowl inversion energy measurement In a J-Young tube, 0.5 mg of sample was dissolved in tetralin (freshly distilled from sodium) (10 ml) under Ar atmosphere. The mixture was then degassed and sealed. The mixture was immersed into a digital controlled oil bath, which was preheated to 219 °C. A corrected mercury thermometer corrected the temperature. The internal temperature (reaction mixture) was measured to be 215 °C (488 K). During heating, samples were taken out for chiral HPLC analysis at 6 h, 12 h, 24 h, 36 h, 60 h and 84 h (HPLC conditions: Daicel Chiralpak IA column, 250 mm × 4.6 mm, hexane/CH 2 Cl 2 / i -PrOH=84.5/15/0.5, flow rate 0.5 ml min −1 , Ultraviolet detector wavelength 321 nm, CD detector wavelength 352 nm, T =10 °C). The selected HPLC charts were shown in the Fig. 4c . Bowl inversion process follows the equation (1) (see Supplementary Methods ): where a is the initial concentration of ( C )-(−)- 1 , assigned as 1, x is the concentration of gradually generated ( A )-(+)- 1 at time t , and k is the inversion rate constant. k= 1.24×10 −6 s −1 ( Fig. 4d ). Bowl inversion energy ΔG ‡ =RTln(k B T h −1 k −1 )=42.2 kcal per mole. Half-lifetime at 488 K: t 1/2 =(ln2)/2 k =77.6 h; Half-life time at 293 K, t 1/2 =54 billion years. Calculation method The optimization of the bowl and flat structures of 1 ( Supplementary Figs S4 and S5; Supplementary Table S3 and S4 ) was carried out using the Gaussian 09 program, using density functional theory calculation at B3LYP/6-311+G (d,p) level of theory [35] . The flat structure has been characterized as the transition state with one imaginary frequency corresponding to the bowl inversion for 1 . The bowl inversion energy was calculated from the difference of the zero-point-corrected energies of the bowl structure and the flat structure. How to cite this article: Tan, Q. et al . Enantioselective synthesis of a chiral nitrogen-doped buckybowl. Nat. Commun. 3:891 doi: 10.1038/ncomms1896 (2012).